Exchange catalysis by tapasin exploits conserved and allele-specific features of MHC-I molecules The repertoire of peptides presented by major histocompatibility complex class I (MHC-I) molecules on the cell surface is tailored by the ER-resident peptide loading complex (PLC), which contains the exchange catalyst tapasin. Tapasin stabilizes MHC-I molecules and promotes the formation of stable peptide-MHC-I (pMHC-I) complexes that serve as T cell antigens. Exchange of suboptimal by high-affinity ligands is catalyzed by tapasin, but the underlying mechanism is still elusive. Here we analyze the tapasin-induced changes in MHC-I dynamics, and find the catalyst to exploit two essential features of MHC-I. First, tapasin recognizes a conserved allosteric site underneath the α 2-1 -helix of MHC-I, ‘loosening’ the MHC-I F-pocket region that accomodates the C-terminus of the peptide. Second, the scoop loop 11–20 of tapasin relies on residue L18 to target the MHC-I F-pocket, enabling peptide exchange. Meanwhile, tapasin residue K16 plays an accessory role in catalysis of MHC-I allotypes bearing an acidic F-pocket. Thus, our results provide an explanation for the observed allele-specificity of catalyzed peptide exchange. Major Histocompatibility Complex class I (MHC-I) molecules present peptide antigens on the surface of nucleated cells for immune surveillance, allowing CD8 + cytotoxic T-lymphocytes to eliminate infected or cancerous cells [1] . Selective loading of peptides derived from the cellular proteome to nascent MHC-I molecules requires the action of the peptide loading complex (PLC) in the endoplasmic reticulum (ER), which consists of the chaperone tapasin, the oxidoreductase ERp57, calreticulin and the transporter associated with antigen processing (TAP) [2] . Tapasin, a key constituent of the PLC, bridges nascent MHC-I heterodimers with the peptide pool delivered by the TAP1/TAP2 heterodimer and catalyzes the peptide editing of MHC-I molecules [3] , [4] , [5] , [6] . TAPBPR (TAP-binding protein-related protein), a homolog of tapasin, can also catalyze the peptide editing of MHC-I molecules but independent of the PLC, thereby providing a second quality control step for efficient loading of antigen [7] , [8] , [9] , [10] , [11] , [12] , [13] , [14] . The single-particle cryo-electron microscopy (cryo-EM) structure of the native PLC provides critical insights into the overall architecture of this molecular machinery and shows that the F-pocket region (α 2-1 -helix and β-strands 7-8) of the MHC-I peptide binding groove is clamped by the N-terminal domain of tapasin [15] . However, the “scoop loop” (loop 11–20 connecting β-strands 1–2 of tapasin), which is hypothesized to interact with the critical F-pocket region of MHC-I, is neither resolved in this structure nor in the crystal structure of tapasin in complex with ERp57 [15] , [16] . Crystal structures of the TAPBPR-MHC-I complex revealed that the corresponding “scoop loop” (loop 22-36 connecting β-strands 1–2) of TAPBPR remodels the peptide binding groove of the MHC-I in the region of the α 2-1 helix, thereby promoting peptide dissociation and subsequently stabilizing the peptide receptive conformation of MHC-I [17] , [18] , [19] , [20] . Furthermore, the TAPBPR scoop loop was also suggested to act as a kinetic trap that lowers the affinity requirements for peptide binding but also prevents dissociation of high-affinity ligands under conditions of limiting peptide [21] . Interestingly, the scoop loop 11–20 in tapasin is considerably shorter compared to the corresponding loop in TAPBPR, leading to the question whether tapasin and TAPBPR engage similar or distinct molecular mechanisms to foster peptide exchange. MHC-I proteins are highly polymorphic and display conformational dynamics in their peptide binding groove [22] , [23] , [24] , [25] , [26] , which confers differential dependence on tapasin or TAPBPR for efficient peptide editing and cell surface expression [5] , [8] , [27] , [28] , [29] , [30] , [31] , [32] , [33] , [34] . The F-pocket of MHC-I, which accommodates the C-terminus of the bound peptide, is critical for MHC-I stability and peptide binding and displays high allelic variation [35] , [36] . The leucine side chain of a murine tapasin scoop-loop-derived linear peptide was observed to anchor to the F-pocket of H2-D b devoid of two C-terminal residues of the antigen [37] . This raises the question whether the interplay of the tapasin loop 11–20 with MHC-I polymorphic regions relates to the observed allele-specific binding and catalysis of tapasin. Here we investigate dynamic changes of MHC-I in the presence of tapasin by NMR spectroscopy and observe conformational dynamics affected by tapasin binding in two regions of the MHC-I molecule. We then address the role of individual residues of the loop 11–20 for tapasin-catalyzed peptide exchange in vitro and define the critical role of tapasin residues L18 and K16 for tapasin allele-specific activity. Our results thus uncover an allele-specific function of the tapasin scoop loop 11– 20 in antigen presentation. Dynamic changes of MHC-I upon shifting into a peptide-receptive state To better understand the peptide-editing process of MHC-I, we investigated the dynamic properties of MHC-I in complex with a photocleavable peptide (pMHC-I), and then followed the changes upon UV exposure by NMR spectrometry. 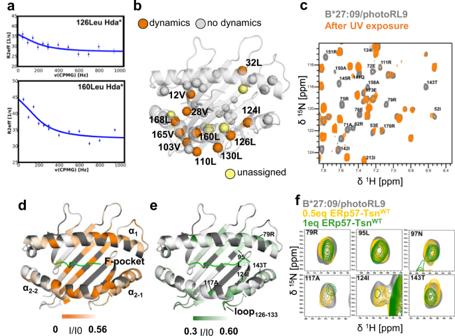Fig. 1: Tapasin “loosens” C-terminus of bound peptide in the pMHC-I. aRepresentative relaxation dispersion curves of B*27:09/photoRL9 methyl groups undergoing conformational exchange (\({R}_{2}^{{eff}}\,\)> 2 s−1) in1H-13C methyl-CPMG experiments recorded at 27 °C at a1H field of 700 MHz. The effective transverse relaxation rate (\({R}_{2}^{{eff}}\)) is shown as a function of the CPMG pulse frequency (νCPMG) for selected methyl groups. Errors were estimated based on duplicate measurements.bResidues showing μs-ms dynamics derived from methyl-CPMG experiments of B27:09/photoRL9 (170 μM) are highlighted as orange spheres in the structure of B*27:09. Other assigned ILV methyl residues which did not show dynamics are mapped as gray spheres. Unassigned residues are shown in light yellow.cZoom view of1H-15N TROSY-HSQC spectra of B*27:09/photoRL9 before (gray) and after UV exposure (orange). Peaks vanished upon UV exposure are labeled.dPeak intensity ratio (Iuv-exposed/Ino-uv) of cleaved B*27:09/photoRL9 (Iuv-exposed) relative to non-cleaved B*27:09/photoRL9 (Ino-uv) is mapped as B-factor in the structure of B*27:09 heavy chain. The range of the intensity ratio is from 0 (orange) to the average Iuv-exposed/Ino-uv(0.58, white). Unassigned residues are colored in dark gray.ePeak intensity ratio (I/I0) of B*27:09/photoRL9 in the presence of ERp57-TsnWT(I) relative to B*27:09/photoRL9 alone (I0) is mapped as B-factor in the structure of B*27:09 heavy chain. The range of the intensity ratio is from half (0.30, forest) to the average I/I0 (0.6, white). Unassigned residues are colored in dark gray.fRepresentative peaks of residues lining the F-pocket showing reduced signal in the presence of ERp57-TsnWT(0.5eq in yellow, 1eq in forest). First, we characterized the dynamics of the human allotype B*27:09 in complex with the photoRL9 peptide (peptide sequence is listed in Supplementary Table 1 ) by 1 H- 13 C multiple-quantum Carr-Purcell-Meiboom-Gill (CPMG) relaxation dispersion NMR experiments. The methyl groups of isoleucine, leucine and valine residues in the MHC-I heavy chain were 1 H- 13 C-labeled. This method allows to detect conformational exchange of the main conformation with sparsely populated states on the micro- to milliseconds (µs-ms) timescale. Indeed, we could observe a relatively large number of methyl-group containing residues exerting conformational exchange and these residues are mainly in the binding groove and polarized towards the α 2 -helix side of it (Fig. 1 a, b ). Subsequently we followed the dynamics features of the complex after peptide cleavage. UV exposure of the photoRL9 peptide results in a 7-mer and a dipeptide fragment. 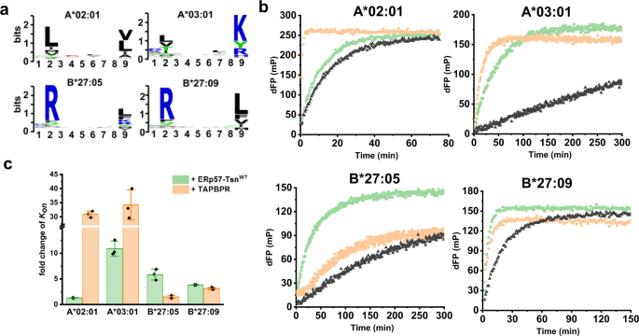Fig. 2: The susceptibility of MHC-I allotypes to tapasin-mediated peptide exchange is different. aSequence logo of peptide that binds to A*02:01, A*03:01, B*27:05, and B*27:09. Peptides known to bind to these alleles were downloaded from IEDB and sequence logos were generated inhttps://weblogo.berkeley.edu.bRepresentative peptide exchange profiles of 500 nM A*02:01/photoKV9, A*03:01/photoKK9, B*27:05/photoRL9, B*27:09/photoRL9 in the absence (black) and presence of equimolar amounts of ERp57-TsnWT(light green) or TAPBPR (wheat) after UV exposure. Peptide exchange was monitored after adding the FITC-version of the peptide used in refolding for each allotype (FITC-GV9 for A*02:01, FITC-KK9 for A*03:01 and FITC-RL9 for B*27:09/05). The measuring time was different for each allotype. dFP means the baseline was subtracted.cThe fold changes of observed association rateKonin the presence of ERp57-TsnWTor TAPPBR for four allotypes. Error bars (standard deviation, SD) were calculated from three independent experiments. The melting temperature T m of the cleaved B*27:09/photoRL9 was lower than that of the intact pMHC-I (Supplementary Table 2 ). Mass spectrometry analysis showed that the 7-mer fragment remains bound to the binding groove of B*27:09 after UV exposure (Supplementary Fig. 1a ). The 1 H- 15 N TROSY-HSQC spectrum of cleaved B*27:09/photoRL9 was recorded and compared with that of the non-cleaved B*27:09/photoRL9 (Supplementary Fig. 1b ). Fig. 1: Tapasin “loosens” C-terminus of bound peptide in the pMHC-I. a Representative relaxation dispersion curves of B*27:09/photoRL9 methyl groups undergoing conformational exchange ( \({R}_{2}^{{eff}}\,\) > 2 s −1 ) in 1 H- 13 C methyl-CPMG experiments recorded at 27 °C at a 1 H field of 700 MHz. The effective transverse relaxation rate ( \({R}_{2}^{{eff}}\) ) is shown as a function of the CPMG pulse frequency (ν CPMG ) for selected methyl groups. Errors were estimated based on duplicate measurements. b Residues showing μs-ms dynamics derived from methyl-CPMG experiments of B27:09/photoRL9 (170 μM) are highlighted as orange spheres in the structure of B*27:09. Other assigned ILV methyl residues which did not show dynamics are mapped as gray spheres. Unassigned residues are shown in light yellow. c Zoom view of 1 H- 15 N TROSY-HSQC spectra of B*27:09/photoRL9 before (gray) and after UV exposure (orange). Peaks vanished upon UV exposure are labeled. d Peak intensity ratio ( I uv- exposed / I no-uv ) of cleaved B*27:09/photoRL9 ( I uv-exposed ) relative to non-cleaved B*27:09/photoRL9 (I no-uv ) is mapped as B-factor in the structure of B*27:09 heavy chain. The range of the intensity ratio is from 0 (orange) to the average I uv-exposed /I no-uv (0.58, white). Unassigned residues are colored in dark gray. e Peak intensity ratio (I/I0) of B*27:09/photoRL9 in the presence of ERp57-Tsn WT (I) relative to B*27:09/photoRL9 alone (I0) is mapped as B-factor in the structure of B*27:09 heavy chain. The range of the intensity ratio is from half (0.30, forest) to the average I/I0 (0.6, white). Unassigned residues are colored in dark gray. f Representative peaks of residues lining the F-pocket showing reduced signal in the presence of ERp57-Tsn WT (0.5eq in yellow, 1eq in forest). Full size image Upon UV exposure, resonances of residues in the binding groove underwent either (i) chemical shift changes (ii) line broadening that is indicative of dynamics in the time range of µs-ms or (iii) both (Fig. 1 c, d and Supplementary Fig. 1b ). Chemical shift changes, which indicate an altered chemical environment due to the dissociation of the C-terminal dipeptide or rearrangement of residues that constitute the peptide and MHC-I interface, were observed throughout the binding groove (Supplementary Fig. 1c , upper chart). Line-broadened resonances, which indicate altered dynamics, were observed throughout the binding groove as well (Supplementary Fig. 1c , lower chart). In particular, residues which are part of the architecture of the F-pocket, including T143, which forms a hydrogen bond with the C-terminus of the peptide, residues L95, N97, and A117 at the bottom of the F-pocket of MHC-I as well as residues R75, E76, D77, and R79, from the α 1 -helix in the F-pocket region, showed strong line broadening (Fig. 1c ), indicating altered dynamics of this region upon UV exposure. In addition to the F-pocket region, heavy chain residues 151–155 that are located close to the central part of the peptide, are also strongly affected, indicating that the altered dynamics extended towards the middle of the binding groove. In contrast, none of the assigned residues in the α 3 domain showed significant signal reduction or chemical shift changes (Supplementary Fig. 1c ). Furthermore, line-broadened peaks re-appeared in the spectrum when the UV-cleaved B*27:09/photoRL9 was incubated with the intact RL9 peptide and the recovered spectrum looks the same as the 1 H- 15 N TROSY-HSQC spectrum of B*27:09/RL9 indicating MHC-I molecules to reversibly adopt a peptide-receptive conformation upon UV exposure. Thus, our data indicates that the release of the C-terminal dipeptide fragment in the F-pocket upon UV exposure turns B*27:09/photoRL9 into a peptide-receptive state, featured by structural and dynamic changes in the binding groove, especially changes in the F-pocket region of the pMHC-I. Interaction with tapasin promotes pMHC-I to adopt a peptide-receptive state We then aime at revealing structural and dynamic changes in pMHC-I complexes induced in the presence of the peptide editor tapasin. Since tapasin alone to enhance peptide loading shows low efficiency [4] , [38] , [39] , tapasin was co-expressed with ERp57 as a conjugate to maintain its full function [4] . Studies showed peptide exchange can be enhanced in vitro by ERp57-Tsn conjugate [16] , [40] , or by Tsn when linked to the heavy chain to increase the affinity [6] . In our system, ERp57-Tapasin conjugate (wild-type, referred to as ERp57-Tsn WT ) can catalyze peptide exchange of non-cleaved B*27:09/photoRL9, although slowly (Supplementary Fig. 2a ). Thus, we added stoichiometric amount of ERp57-Tsn WT to intact B*27:09/photoRL9, to mimic the interaction between tapasin and suboptimal-peptide-loaded-MHC-I within the PLC and subsequently recorded the 1 H- 15 N TROSY-HSQC spectrum. While almost no chemical shift changes could be seen (Supplementary Fig. 2b ), line-broadened resonances of residues in the peptide binding groove were observed (Fig. 1e , Supplementary Fig. 2b ). Interestingly, many of these resonances (e.g. R79, N97, A117, D120, I124, T143, A151, Fig. 1f ) overlapped with those affected by UV exposure (compare Fig. 1d , e and Supplementary Fig. 2b ), although not as strongly as in the UV exposed spectrum. In particular, signal intensity of F-pocket residue T143 is significantly attenuated, together with other F-pocket residues N97, A117 (Fig. 1f ), indicating that tapasin-induced altered F-pocket dynamics similar to the features seen for the pMHC-I molecule devoid of the C-terminal dipeptide after UV- exposure. Thus, we suggest that tapasin promotes pMHC-I to adopt a receptive state by affecting the residues in the F-pocket that interact with the C-terminus of the peptide, facilitating release of bound peptide and eventually exchanged by an incoming competitor peptide. In addition to the F-pocket region, residues in the loop 126-133 connecting strands β7-β8, were also significantly affected by addition of ERp57-Tsn WT (Supplementary Fig. 2d ), which is in line with the observed interaction between this region with the hairpin loop 187– 196 (loop connecting β-strands 9–10) of tapasin in the cryo-EM structure of the PLC (Supplementary Fig. 2c ) [15] . Notably, I124, L126 and L130, close or within the loop 126-133 that was affected by tapasin binding, also showed conformational exchange dynamics in the intact pMHC-I complex (Fig. 1b ), suggesting that an alternative conformation of this loop might pre-exist in solution and could be recognized by tapasin. Indeed, mutations of residues (D128, W133) within the loop 126-133 have been previously shown to affect the MHC-I interaction with tapasin and it was suggested that the conformation of the loop 126-133 might be modulated by tapasin [41] . Thus, the loop 126-133 represents an important region for complex formation. There are also some important differences between tapasin-induced and UV-exposure-induced changes in MHC-I. While individual residues of the F-pocket clearly indicate changes at the site of interaction with the C-terminus of the peptide in both cases, a full destabilization of the α 2-1 -helix is only observed after UV exposure. Influence of ERp57-Tsn on peptide exchange kinetics Although the peptide exchange of un-cleaved B*27:09/photoRL9 can be enhanced in the presence of ERp57-Tsn WT (Supplementary Fig. 2a ), the association rate was extremely slow, and we thus decided to perform subsequent experiments under conditions of UV exposure. To be able to draw more general conclusions, we performed our analysis with two allotypes, B*27:09 and B*27:05, which only differ at position 116 (H116 and D116, respectively), and two pre-bound photocleavable (photoRL9 and photoIF9) as well as two incoming peptides (FITC-RL9 and FITC-IF9). The photoRL9 has a significantly higher predicted affinity than photoIF9 for B*27:09 as well as B*27:05 (Supplementary Table 1 ). To indirectly obtain the affinities of the cleaved peptide for MHC-I variants we compared the thermostability of the four combinations of allotypes and pre-bound peptides after peptide cleavage. We observed a 6 and 2 °C higher stability of the B*27:09 and B*27:05 in complex with photoRL9 compared to photoIF9, respectively (Supplementary Fig. 3a ). This indicates a correspondingly higher affinity of the cleaved photoRL9 (7-mer) to the complexes. Peptide exchange kinetics were then monitored by adding the fluorescent-labeled versions of the corresponding peptides directly after UV-cleavage, either in the absence or presence of equimolar ERp57-Tsn WT (Supplementary Fig. 3b–e ). The uncatalyzed peptide exchange rate ( K on ) was higher for the less stable cleaved photoIF9 complexes (Supplementary Fig. 3f ) while the enhancements of the K on by ERp57-Tsn WT for both allotypes were larger in case the higher affinity peptide photoRL9 was used as pre-bound peptide (Supplementary Fig. 3g ). In contrast, the affinity of the incoming peptide affects the enhancement of K on by ERp57-Tsn WT to a lower extend when the allotype is in complex with the same photocleavable peptide (Supplementary Fig. 3g ). These results are in line with the previous finding obtained with the B*44:02 allotype that showed tapasin to catalyze thermodynamically favored but kinetically disfavored exchange of suboptimal peptides for high-affinity peptides [40] . Allotypic differences in tapasin-catalyzed peptide exchange in vitro It has been shown that the F-pocket region of pMHC-I is important for its tapasin dependence [32] . When we compared the tapasin-induced fold change of K on of B*27:05 with B*27:09 using the same pre-bound and incoming peptides, B*27:05 is found to be more susceptible to tapasin-mediated peptide exchange than B*27:09 (Supplementary Fig. 3g ). To delineate how the F-pocket architecture more generally correlates with its tapasin dependence we extended our analysis to two HLA-A allotypes. The allotype A*02:01 comprises a hydrophobic F-pocket with Y116 forming the floor while A*03:01 contains an Asp at this position, as it is in B*27:05. The charged surface area of the individual allotypes’ F-pocket is displayed in Supplementary Fig. 4a . Clearly, the F-pocket of these four allotypes shows a gradient in acidity: A*03:01 > B*27:05 > B*27:09 > A*02:01, in line with a differential preference for basic or hydrophobic residues at the C-terminus (PΩ) of bound peptides (Fig. 2a ). Fig. 2: The susceptibility of MHC-I allotypes to tapasin-mediated peptide exchange is different. a Sequence logo of peptide that binds to A*02:01, A*03:01, B*27:05, and B*27:09. Peptides known to bind to these alleles were downloaded from IEDB and sequence logos were generated in https://weblogo.berkeley.edu . b Representative peptide exchange profiles of 500 nM A*02:01/photoKV9, A*03:01/photoKK9, B*27:05/photoRL9, B*27:09/photoRL9 in the absence (black) and presence of equimolar amounts of ERp57-Tsn WT (light green) or TAPBPR (wheat) after UV exposure. Peptide exchange was monitored after adding the FITC-version of the peptide used in refolding for each allotype (FITC-GV9 for A*02:01, FITC-KK9 for A*03:01 and FITC-RL9 for B*27:09/05). The measuring time was different for each allotype. dFP means the baseline was subtracted. c The fold changes of observed association rate K on in the presence of ERp57-Tsn WT or TAPPBR for four allotypes. Error bars (standard deviation, SD) were calculated from three independent experiments. Full size image Peptide exchange experiments were performed by adding the FITC-version of the high-affinity peptides used in refolding for each allotype after UV exposure. The peptide affinity and thermal stability data of the corresponding photo-MHC-I molecules are listed in Supplementary Table 1 and 2 , respectively. After UV exposure, in the presence of ERp57-Tsn WT , the peptide exchange rate was increased 10.89 ± 1.48 fold for A*03:01, 5.83 ± 1.06-fold for B*27:05, 3.83 ± 0.07-fold for B*27:09, 1.31 ± 0.08-fold for A*02:01 (Fig. 2c ). ERp57-Tsn WT slightly accelerates the peptide exchange of A*02:01 (Fig. 2 b, c ) and similar results were obtained for other high-affinity FITC-labeled peptides (Supplementary Fig. 4b , c), which is in agreement with previous studies showing that refolding of A*02:01 can be facilitated by tapasin [42] . Thus, our data indicate that susceptibility to tapasin-mediated peptide exchange of human allotypes appears to be positively correlated with the gradient of acidity of the MHC-I F-pocket. 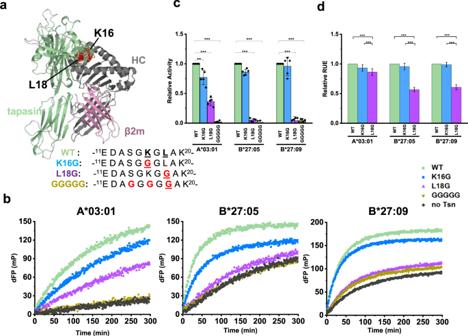Fig. 3: The role of tapasin scoop loop11–20in mediating peptide exchange of MHC-I. aThe loop11–20of tapasin in the modeled MHCI-ERp57-Tsn complex (ERp57 is not shown here). Residue 16 and 18 were colored red. The sequence of tapasin scoop loop11–20mutants are shown besides.bRepresentative peptide exchange profiles of 500 nM A*03:01/photoKK9, B*27:05/photoRL9, B*27:09/photoRL9 in the absence (black) and presence of equimolar amounts of ERp57-TsnWT(light green), ERp57- TsnL18G(sky blue), ERp57-TsnK16G(purple), and ERp57-TsnGGGGG(golden). FITC-KK9 for A*03:01 and FITC-RL9 for B*27:05. FTIC-IF9 (IRAAKFITCPPLF) was used for better resolution of the kinetics for B*27:09. dFP means the baseline was subtracted.cRelative catalytic activity of ERp57-Tsn loop11–20mutants compared to ERp57-TsnWTtowards three allotypes. The observed association rates (Kon_Tsn_mutant) were determined for each mutant on the corresponding MHC-I allotype and relative activity was calculated by the formula of (Kon_Tsn_mutant– Kon_Tsn-)/(Kon_Tsn_WT–Kon_ Tsn-). Error bar (SD) was calculated from five independent experiments.dNormalized free energy values of the modeled tapasin mutants calculated in Rosetta Energy Unit (REU). Error bar (SD) was calculated from 100 data points. Inccomparison of loop mutants to WT, the two-sample unequal variance Student’sttest was performed, indmean comparison method is Tukey, *p< 0.05, **p< 0.01, ***p< 0.001. We then generated F-pocket mutants of A*02:01, A*03:01, and B*27:05 to probe the positive correlation between tapasin enhancement on peptide exchange and the acidity of the F-pocket (F-pocket mutants are listed in Supplementary Table 3 ). Indeed, the peptide exchange rates of B*27:05H114R and B*27:05D116Y refolded with photoRL9 was less enhanced by tapasin than that of B*27:05WT (Supplementary Fig. 4d, e , the acidity of the F-pocket is: B*27:05WT > B*27:05D116Y > B*27:05H114R). A similar trend was observed for the F-pocket mutants of A*03:01 (Supplementary Fig. 4f–h ). In this case the FITC-KK9 used for monitoring peptide association of A*03:01WT had to be replaced by FITC-KV9-2 (sequence is listed in Supplementary Table 3 ) for A*03:01D116Y and A*03:01R114H/D116Y mutants due to the low affinity of FITC-KK9 for these two mutants. A comparison of the peptide exchange of these two F-pocket mutants showed less tapasin dependence for A*03:01D116Y compared to that of A*03:01R114H/D116Y, which is in line with the acidity gradient of the mutants F-pocket (Supplementary Fig. 4f–h ). In the case of the A*02:01 allotype, no significant tapasin enhancement was observed for the A*02:01Y116D mutant or the A*02:01H114D mutant (Supplementary Fig. 4i–k ), indicating that the intrinsically low dependence on tapasin cannot be further enhanced by acidification of the F-pocket in this case. In addition, we performed peptide exchange experiments with TAPBPR. In the presence of TAPBPR (Fig. 2b ), peptide exchange rates of A*02:01, A*03:01, B*27:09, and B*27:05 were increased by 30.9 ± 1.12, 34.28 ± 5.3, 3.13 ± 0.23, and 1.48 ± 0.23-fold, respectively (Fig. 2c ), which is in line with previous reports that TAPBPR has a strong preference for HLA-A alleles [28] . It is worth noting that in our experimental set up B*27:09 is more TAPBPR susceptible than B*27:05. This is in accord with a previous report where in the presence of TAPBPR no significant enhancement of peptide binding for B*27:05 was detected, while for B*27:09 an enhancement of more than 100% was observed [28] . We then ask the question which structural or dynamic features of tapasin could explain the observed different susceptibility to tapasin-catalyzed peptide exchange for different allotypes. L18 is the key residue in the scoop loop 11– 20 of tapasin to mediate peptide exchange of MHC-I In the current cryo-EM PLC structure, residues within the tapasin scoop loop 11–20 which are close to the F-pocket of MHC-I are not resolved, nor in the crystal structure of ERp57-Tsn conjugate alone, hinting at an increased flexibility of this region. We then used the cryo-EM structure of the PLC (PDB ID 6ENY) as a scaffold to model an ensemble of MHC-I-ERp57-Tsn complex structures to illustrate potential conformations of loop 11–20 of tapasin (Fig. 3a ). To test the potential function of this scoop loop for tapasin catalytic activity, we mutated the two amino acids K16 and L18 that have a side-chain conceivably long enough to reach into the F-pocket (Fig. 3a ). Glycine was chosen as a substitute to allow for maximum flexibility of the loop, potentially allowing the residues at position 16 or 18 to reach into the F-pocket. As a control, the hypothetically fully inactive mutant ERp57-Tsn GGGGG was also included. The stability of mutants was similar to ERp57-Tsn WT (Supplementary Fig. 5 ). Since the peptide exchange of A*02:01/photoKV9 was only slightly enhanced by tapasin, we focused on A*03:01, B*27:05, and B*27:09 allotypes and investigated the catalytic activity of the mutants ERp57-Tsn L18G , ERp57-Tsn K16G and ERp57-Tsn GGGGG on peptide exchange. The relative catalytic activity of the mutants compared to the wild type were calculated by the formula ((K on_Tsn_mutant – K on_Tsn - )/(K on_Tsn_WT – K on_ Tsn - ) for each allotype. Fig. 3: The role of tapasin scoop loop 11– 20 in mediating peptide exchange of MHC-I. a The loop 11– 20 of tapasin in the modeled MHCI-ERp57-Tsn complex (ERp57 is not shown here). Residue 16 and 18 were colored red. The sequence of tapasin scoop loop 11– 20 mutants are shown besides. b Representative peptide exchange profiles of 500 nM A*03:01/photoKK9, B*27:05/photoRL9, B*27:09/photoRL9 in the absence (black) and presence of equimolar amounts of ERp57-Tsn WT (light green), ERp57- Tsn L18G (sky blue), ERp57-Tsn K16G (purple), and ERp57-Tsn GGGGG (golden). FITC-KK9 for A*03:01 and FITC-RL9 for B*27:05. FTIC-IF9 (IRAAK FITC PPLF) was used for better resolution of the kinetics for B*27:09. dFP means the baseline was subtracted. c Relative catalytic activity of ERp57-Tsn loop 11– 20 mutants compared to ERp57-Tsn WT towards three allotypes. The observed association rates ( K on_Tsn_mutant ) were determined for each mutant on the corresponding MHC-I allotype and relative activity was calculated by the formula of ( K on_Tsn_mutant – K on_Tsn - )/ (K on_Tsn_WT – K on_ Tsn - ) . Error bar (SD) was calculated from five independent experiments. d Normalized free energy values of the modeled tapasin mutants calculated in Rosetta Energy Unit (REU). Error bar (SD) was calculated from 100 data points. In c comparison of loop mutants to WT, the two-sample unequal variance Student’s t test was performed, in d mean comparison method is Tukey, * p < 0.05, ** p < 0.01, *** p < 0.001. Full size image As shown in Fig. 3b , the activity of ERp57-Tsn L18G in catalyzing the peptide exchange of these three allotypes was strongly reduced (0.36 ± 0.06 for A*03:01, 0.05 ± 0.02 for B*27:05, and 0.04 ± 0.06 for B*27:09, Fig. 3c , purple bars), indicating that L18 is critical for tapasin catalytic activity. In contrast to that, the catalytic activity of ERp57-Tsn K16G on peptide exchange was 0.77 ± 0.12 for A*03:01, 0.86 ± 0.05 for B*27:05, and 0.95 ± 0.15 for B*27:09 (Fig. 3c , blue bars), displaying a negative correlation to the gradient of acidity of the allotypes’ F-pocket. Expectedly, the catalytic activity of ERp57-Tsn GGGGG on peptide exchange for all allotypes was completely abolished (0.01 ± 0.01 for A*03:01, 0.02 ± 0.01 for B*27:05 and 0.03 ± 0.02 for B*27:09, Fig. 3c , golden bars). Taken together, for B*27:05 and B*27:09, the activity of ERp57-Tsn was nearly abolished by the L18G mutation, resulting in a peptide exchange rate nearly equal to that of uncatalyzed MHC-I (black curve, Fig. 3b ), while the K16G mutation did not significantly impair the activity of ERp57-Tsn. Thus, for the B*27:05 and B*27:09 allotypes, L18 but not K16 appears to be important for tapasin catalytic activity. Different to B*27:05 and B*27:09, the peptide exchange of A*03:01 was still enhanced by ERp57-Tsn L18G (Fig. 3b ), indicating that K16 can rescue the activity of ERp57-Tsn L18G for A*03:01 to a certain extent. Concomitantly, ERp57-Tsn K16G showed significantly reduced activity (0.73 ± 0.12) for A*03:01, suggesting that K16 is important for the catalytic activity of tapasin in case of the A*03:01 allotype. Additionally, we calculated the Rosetta Energy Scores (REU) of the MHC-I-ERp57-Tsn complex models with the desired scoop loop mutation for each allotype [43] , [44] , [45] . The REU were averaged for all generated models per mutant. As shown in Fig. 3d , the relative REU (rREU) of all three MHC-I allotypes in complex with ERp57-Tsn K16G was only slightly reduced as compared to ERp57-Tsn WT (0.93 ± 0.05 for A*03:01, 0.95 ± 0.05 for B*27:05, and 0.98 ± 0.03 for B*27:09), suggesting a marginal impact of the K16G mutation on overall complex stability. In contrast, rREU of the MHC-I -ERp57-Tsn L18G complex was reduced to 0.56 for B*27:09 and 0.60 for B*27:05, indicating the important role of L18 to stabilize these complexes. Interestingly, rREU of A*03:01-ERp57-Tsn L18G was still 0.86 that of wild type, again indicating that L18 is not the only important residue for stabilization of this allotype. Taken together, our data highlight the critical role that L18 plays for tapasin catalytic activity while K16 plays an auxiliary role that is of importance for allotypes bearing an acidic F-pocket as exemplified here by A*03:01. The role of K16 in the loop 11– 20 is dependent on the F-pocket nature of MHC-I molecules In order to unravel the relevance of the tapasin loop 11–20 for the tapasin catalytic activity on MHC allotypes that differ in the chemical nature of their F-pocket, we designed several tapasin mutants with different combinations of leucine or lysine at positions 16 and 18 of the loop 11– 20 : K16L (SGLGL), L18K (SGKGK), GGGGL, GGGGK, GGLGG, and GGKGG (sequences are listed in Fig. 4a , stability data was listed in Supplementary Fig. 5 ). The A*03:01 allotype bearing the most acidic F-pocket (preference for basic residues) and B*27:09 bearing the least acidic F-pocket (preference for hydrophobic residues) were chosen to test the catalytic activity of these tapasin mutants. Fig. 4: The role of K16 is the F-pocket nature dependent. a The sequence of Tsn loop 11– 20 mutants . b , c upper panel: Relative activity of tapasin loop 11– 20 mutants to catalyze peptide exchange compared to ERp57-Tsn WT towards A*03:01 and B*27:09. FTIC-KK9 was used for A*03:01, FTIC-IF9 (IRAAK FITC PPLF) was used for better resolution of B*27:09. Error bars (SD) were calculated from three independent experiments. For comparison of loop mutants to WT, the two-sample unequal variance Student’s t test was performed (* p < 0.05, ** p < 0.01, *** p < 0.001). Lower panel: Representative peptide exchange profiles of 500 nM A*03:01/photoKK9, and B*27:09/photoRL9 in the absence (black) and presence of equimolar amounts of tapasin loop mutants. dFP means the baseline was subtracted. These curves were recorded on the PerkinElmer VICTOR 3 V machine. Full size image As can be seen in Fig. 4 b, c , the ERp57-Tsn K16L mutant showed no significantly different catalytic activity compared to ERp57-Tsn WT for A*03:01 (0.93 ± 0.16 of WT) and increased catalytic activity for B*27:09 (1.26 ± 0.06 of WT). While ERp57-Tsn L18K displayed no activity for both allotypes. The relative activity of ERp57-Tsn GGGGL was 0.40 ± 0.12 for A*03:01 and 0.77 ± 0.14 for B*27:09, while the relative catalytic activity of ERp57-Tsn GGGGK was 0.23 ± 0.05 for A*03:01 and showed no catalytic activity for B*27:09. However, ERp57-Tsn GGKGG and ERp57-Tsn GGLGG showed an opposite behavior in catalysing peptide exchange of A*03:01 and B*27:09: ERp57-Tsn GGKGG can enhance peptide exchange of A*03:01 as efficiently as ERp57-Tsn WT , while ERp57-Tsn GGLGG can only slightly enhance the peptide exchange of A*03:01 (with 0.35 ± 0.05, the activity was similar to that observed for ERp57-Tsn L18G , 0.36 ± 0.05 of WT). In contrast, ERp57-Tsn GGKGG was not able to promote peptide exchange of B*27:09 at all, while the activity of ERp57-Tsn GGLGG on B*27:09 was the same as ERp57-Tsn WT . These results indicate that the exact position of K16 and critical L18 residues is malleable to a certain extent and the contribution of K16 is distinct for the two allotypes. The catalytic activity of the ERp57-Tsn K16L mutant, which has two leucine residues in the loop, was slightly higher than ERp57-Tsn WT for B*27:09, suggesting position 16 can contribute to the activity of tapasin, again demonstrating that the role of the residue at position 16 strongly depends on the polarity of the F-pocket and a similar dichotomy was observed for position 18, albeit not as pronounced as for position 16. The opposite activity of ERp57-Tsn GGKGG and ERp57-Tsn GGLGG to catalyze peptide exchange of A*03:01 and B*27:09 suggests that when there is no Leu at position 18, only one Leu or Lys at position 16 in the loop is sufficient for tapasin to maintain its peptide exchange function. The activity of ERp57-Tsn GGLGG was higher than that of ERp57-Tsn GGGGL for B*27:09, demonstrating the importance of the loop’s mobility, indicating that the residue at position 16 can reach into the F-pocket better than Leu in position 18 in the context of a flexible loop. The interaction of ERp57-Tsn mutants with MHC-I indicates critical structural elements Next, in order to investigate if scoop loop mutants differently affect the interaction of tapasin with pMHC-I, we analyzed the affected residues of B*27:09/photoRL9 upon addition of ERp57-Tsn GGLGG and ERp57-Tsn L18G mutants by NMR spectroscopy. Similar to ERp57-Tsn WT , line broadening of a similar number of peaks were observed in the presence of both mutants. The binding groove residues significantly affected by ERp57-Tsn GGLGG and ERp57-Tsn L18G overlapped largely with residues affected by ERp57-Tsn WT (Fig. 5b , the red boxed region). Fig. 5: NMR analysis of tapasin mutants interacting with MHC-I. a Representative zoom view of the overlay of 1 H- 15 N TROSY-HSQC spectra of 50 µM B*27:09/photoRL9 (gray) and in the presence of equimolar ERp57-Tsn WT (green), ERp57-Tsn GGLGG (blue) or ERp57-Tsn L18G (purple). Attenuated peaks are marked. b Peak intensity ratio analysis (I/I0) of B*27:09/photoRL9 in the presence of ERp57-Tsn WT , ERp57-Tsn L18G , ERp57-Tsn GGLGG , and TAPBPR against B*27:09/photoRL9 (I0) are plotted against residue sequence. Significantly reduced residues (below I/I0 average – δ) were highlighted in corresponding dark color. Unassigned residues are plotted as gray bars. Red squared region means affected region in the peptide binding groove in the presence of tapasin or TAPBPR. Black squared region means region only affected by TAPPBR. c Peak intensity ratio (I/I0) are mapped as B-factor on the structure of B*27:09. The range of the intensity ratio is from 0.3 to 0.7 for all mutants. The color code is the same as in b . Unassigned residues are plotted as white color. Full size image Unexpectedly, residue T143 was also affected by adding ERp57-Tsn L18G (Fig. 5a ), which suggests that this mutation in the loop 11– 20 does not significantly affect tapasin interacting with pMHC-I’s F-pocket region, although L18 is critical for the catalytic activity of tapasin. It is well known that T143 as well as Y84 form essential H-bonds with the carboxyl group of the bound peptide in the pMHC-I and we also observed these two H-bonds in the crystal structure of B*27:09/photoRL9 (Supplementary Fig. 6c ). Thus, we hypothesize that the observed signal intensity reduction of T143 (Y84 is not assigned) is indicative of the destabilization of the H-bonds of the F-pocket region in the presence of tapasin. As a comparison, we also analyzed the effect of TAPBPR on residues of B*27:09/photoRL9 by NMR spectroscopy. Similar to tapasin, no chemical shift changes but line broadening of peaks were observed. A stronger intensity reduction in the binding groove of MHC-I was detected in the presence of TAPBPR as compared to tapasin, especially for residues at the bottom of the F-pocket (Fig. 5b ). In addition to residues in the loop 126– 133 , the N-terminus of the α 2-1 -helix was strongly affected by TAPBPR similar to what we observed for the UV-cleaved B*27:09/photoRL9 complex (Fig. 1d ). In contrast to tapasin, peak intensity of residues in the β-sheet 225-232 of the α3-domain of the MHC-I heavy chain were strongly reduced in the presence of TAPBPR (Fig. 5b , black boxed region), which is in line with the observed interaction between the IgG domain of TAPBPR and β-sheet 225-232 of the α3-domain in the crystal structure of the MHC-I-TAPBPR complex [17] , [18] . This clearly suggests that the interaction between the IgG domain of TAPBPR with α3 domain of the heavy chain is stronger compared to tapasin, where we did not observe the corresponding signal loss (Fig. 5b ). Tapasin, a critical component of the PLC, acts as the peptide editor to shape the peptide pool presented by MHC-I on the cell surface. The cryo-EM structure of the PLC provides insight into how tapasin interacts with MHC-I as well as other PLC components. However, the molecular mechanism of tapasin-mediated peptide exchange of MHC-I remains elusive, given the inherent dynamics of critical regions within the complex. Here, we capitalize on NMR analysis to demonstrate that the dynamic properties of residues in the F-pocket are affected by tapasin binding and coincide with residues that underwent changes upon UV-induced peptide cleavage. A recent study reported that the switch between a peptide-free unlocked state and a peptide-bound locked state of the F-pocket is important for peptide binding [36] . Our results indicate that tapasin promotes peptide exchange of pMHC-I by switching the F-pocket to the unlocked state. T143, similar to Y84, forms a hydrogen bond to the terminal carboxylate group of the peptide and the observed line broadening of its NH group in the presence of tapasin (Fig. 1f ) most likely reflects the loss of this H-bond as a consequence of partial peptide dissociation. Interestingly, in a recent MD simulation based on the entire PLC, E72 of tapasin was found to contact the conserved Y84 [46] , [47] , [48] and a E72K mutant shows impaired MHC-I binding compared to wild-type tapasin [16] . In the MHC-I-TAPBPR-structure, E105 which structurally corresponds to E72 in tapasin, is found to form an H-bond with Y84 of the MHC-I molecule, thereby replacing the H-bond formed with the C-terminus of the peptide [17] , [18] . Thus, we conclude that disruption of the C-terminal hydrogen bonds between the conserved residues Y84 and T143 of MHC-I and peptide represents a hallmark of tapasin action. Interestingly, we see NMR signal reduction of T143 in the presence of the catalytically inactive ERp57-Tsn L18G mutant (Fig. 5 ). Thus, it must be concluded that the initial destabilization or even disruption of the hydrogen bonds between the MHC-I molecules and the C-terminus of the peptide are independent of the scoop loop. Unlocking of the F-pocket region conceivably allows the loop 11– 20 of tapasin to place its L18 residue near or into the F-pocket (Fig. 6 ). Fig. 6: The proposed mechanism of tapasin-mediated peptide exchange. Step 1: pMHC-I molecules sample conformations, which determine peptide binding and tapapsin binding. Tapasin recognizes a certain state of pMHC-I by approaching pMHC-I from the α 2 -helix side of the pMHC-I. Interaction between its loop 187-196 with the loop 126-133 of heavy chain provides initial binding which alters the dynamics of the peptide binding groove and subsequently together with the interaction between its E72 in strands β3 and Y84 of the heavy chain promote the C-terminus of peptide to adopt loose binding in the F-pocket accompanied. Now pMHC-I switches to the unlocked state. MHC-I charged with very low affinity peptide can switch to peptide unlocked state automatically by the motion of the bound peptide adopting loose binding state. Step 2: The scoop loop 11-20 interacts with the F-pocket region and stabilize the F-pocket with side chain of L18. Now pMHC-I switches to the peptide receptive state. For allotypes bearing a negatively charged F-pocket, tapasin can also use the residue K16 in the scoop loop 11-20 to stabilize the charged F-pocket, which increases the efficiency of tapasin-mediated peptide exchange. Step 3: The upcoming peptide competes for the F-pocket until the affinity is high enough to replace the side chain. Step 4: Once the high-affinity peptide binds, tapasin is released from the pMHC-I. Full size image In addition to the altered dynamics of the F-pocket, the loop 126– 133 of the heavy chain was also strongly affected by tapasin, as indicated by severe line broadening of residues in this region (Supplementary Fig. 2c ). Interestingly, this loop 126– 133 also shows conformational exchange in the CPMG experiments (Fig. 1b ), indicating that a rare second conformation is already present in stable pMHC-I complexes. The loop 126-133 region was observed to be contacted by the tapasin loop 187– 196 in the PLC structure and mutations in both loops abrogate peptide editing in a cellular setting [15] , [16] , [41] , indicating the possible role of the interaction in forming the complex. Notably, both loops are also highly conserved among species (Supplementary Fig. 7a , b ), implying that they represent an allotype-independent interface. We investigated the function of human tapasin loop 11– 20 in catalyzing peptide exchange of MHC-I in more detail and identified L18 as the critical residue in mediating peptide exchange, which is in line with published studies on the role of Leu both in the tapasin [21] , [37] and TAPBPR scoop loop [20] . Three human allotypes with distinct F-pockets were studied to demonstrate the importance of L18 in all cases. In addition, we found that K16 contributes to the activity of tapasin for MHC-I allotypes bearing an acidic F-pocket. Our mutational studies indicate that the chemical nature as well as flexibility of the loop 11– 20 tunes the catalytic activity of tapasin. The catalytic activity of ERp57-Tsn L18G (SGKGG) was significantly lower than that of ERp57-Tsn GGKGG towards A*03:01, although the only difference is a serine in position 14 of the tapasin loop in ERp57-Tsn L18G , indicating that the presence of a polar residue can also influence the allele-specific tapasin activity, at least for some alleles. We expected to see that the introduction of an additional Lys in position 18 would increase the activity of tapasin for A*03:01, which was not the case here. The reduced activity might be explained by the electrostatic repulsion between K16, K18, and K20 in the ERp57-Tsn L18K loop. As for the allelic differences in tapasin-catalyzed peptide exchange, we showed that the influence of tapasin on peptide association kinetics is positively correlated with the acidity of the F-pocket of the MHC-I, as is shown in detail with B*27:05 and A*03:01 F-pocket mutants (Supplementary Fig. 4d–h ). Our results are consistent with the difference in tapasin dependence of the well-studied allotypes B*44:02 and B*44:05, which differ by only one residue at the bottom of the F-pocket: B*44:02, which harbors an Asp at position 116, is strongly tapasin dependent, while B*44:05, bearing a Tyr at position 116, is of low tapasin dependence. The positive correlation between the acidity of the F-pocket of MHC-I and tapasin enhancement on peptide exchange is also in agreement with results from a recently published paper in which highly tapasin-independent allotypes (e.g., A*68:01, A*02:02, A*02:01, B*81:01, B*35:01, and B*42:01) display hydrophobic F-pockets, while the tapasin-dependent allotypes (e.g., A*01:02, A*01:01, A*36:01, B*44:03, and B*44:02) contain an Asp at position 116 [49] . For the less tapasin-dependent allotype A*02:01, increasing the F-pocket acidity did not enhance tapasin dependence (Supplementary Fig. 4j, k ), suggesting that the scoop loop interaction is not the main determinant for catalytic activity in this case. We explored the peptide exchange rates of B*27:09/05 with different photocleavable peptides for which affinities ranged from high to medium in the presence of Erp57-Tsn WT (Supplementary Fig. 3 ). Our results indicate that the catalytic effect of tapasin is more pronounced when the affinity of the remaining 7-mer peptide is relatively high. In case the 7-mer peptide affinity is low, dissociation will be fast and not require tapasin. The conclusion that tapasin is more efficiently replacing medium-to-high-affinity peptides is in line with a report using a leucine zippered complex of HLA-B*08:01 and tapasin [6] and a study that showed that tapasin catalyzes thermodynamically favored but kinetically disfavored exchange of suboptimal peptide for high-affinity peptides [40] . Tapasin and TAPBPR utilize conserved structural features to allow for the initial steps of catalyzed peptide exchange. Conserved residues (E72 in tapasin corresponding to E105 in TAPBPR) in the catalysts provide an alternative hydrogen bonding pattern for F-pocket residue Y84, thereby facilitating release of the C-terminus of bound peptides. Interestingly, the dynamics of the F-pocket region were also affected by adding TAPBPR (Fig. 5b ), suggesting TAPBPR and tapasin share similar mechanisms to turn MHC-I to a peptide-receptive state by modulating the dynamics in the F-pocket region. The loop 126– 133 region also showed NMR line broadening in the presence of TAPBPR (Fig. 5b ) and the loop 126-133 was observed to form polar contacts with the “jack hairpin” loop of TAPBPR in complex with MHC-I [17] , [18] , implying that both molecules share a common mechanism where the dynamics of the loop 126-133 of MHC-I molecules is sampled by the “jack hairpin” loop of either tapasin or TAPBPR. However, the affected region extends into the structurally proximal α 2-1 helix in TAPBPR (Fig. 5b ) which might reflect the 2 Å displacement of this helix seen upon complex formation [15] , [17] , [18] . Several groups recently have investigated the function of the TAPBPR scoop loop [19] , [20] , [21] , and one of these studies found TAPBPR preferentially promotes peptide exchange of MHC-I allotypes bearing a hydrophobic F-pocket [28] . The authors proposed that L30 in the human TAPBPR loop is the key residue to mediate peptide dissociation [20] . Interestingly, the charge state of the mouse TAPBPR scoop loop is similar in sequence to human TAPBPR (Supplementary Fig. 8a ) in line with the observed hydrophobicity of all mouse MHC-I alleles. In this respect it is interesting that a recent study indicates the long G24-R36 scoop loop of TAPBPR containing the critical leucine does not reach into the F-pocket but rather sits on top of it thereby acting as a kinetic trap for medium-to-high-affinity peptides under conditions where peptide concentrations are low [21] . Thus, while TAPBPR can enhance peptide exchange of high-affinity peptides during MHC complex maturation, it may also chaperone existing complexes along the transport through the ER and Golgi compartments when no high-affinity peptides are available. Based on the finding that tapasin loop composition and flexibility is important for catalysis, we compared the tapasin scoop loop sequence of different species and found that L18 is conserved among species (Supplementary Fig. 8b ). This agrees with our conclusion that L18 is the critical residue to mediate peptide exchange, which is also in line with a previous study showing that mutating Leu in the mouse tapasin loop 11–20 significantly reduced the surface expression level of H2-K b 34 . In contrast to the conserved Leu, there is no Lys in the mouse tapasin scoop loop, which coincides with none of the reported murine MHC-I allotypes to bear an acidic F-pocket. Furthermore, in our experiments the ERp57-Tsn GGGGL mutant serves as a mimic of mouse tapasin and we find its activity to be higher for B27:09 compared to A*03:01 (Fig. 4b, c ). Thus, according to our mechanistic findings, the emergence of a Lys residue in the human tapasin scoop loop is to enhance the catalytic activity of tapasin for human allotypes bearing an acidic F-pocket. Future research will have to show whether a possible co-evolution between tapasin and MHC-I allotypes has occurred in order to enhance the antigenic repertoire and immunological fitness of non-rodent mammalian species. Refolding and purification of pMHC-I proteins Human β 2 m (1-100), the luminal domain of HLA-A*02:01(1-276), HLA-A*03:01(1-274), HLA-B*27:05 (1-277), and HLA-B*27:09 (1-277) were expressed in BL21(DE3) Escherichia coli as inclusion body and purified as described below [50] : Cell pellets were resuspended with P1 lysis buffer (50 mM Tris, 1% (w/v) sodium deoxycholate, 1% (w/v) Triton X-100, 100 mM NaCl, 0.1% (w/v) NaN3, 0.5 mM MgCl 2 , 10 mM DTT, 20 µg/mL DNase I, pH 7.5) and sonicated for 30 min on ice water. The sonicated lysate was centrifuged at the speed of 12,000× g for 10 min and the supernatant was trashed. The white pellet is the inclusion bodies. Inclusion bodies were first washed twice with P2 buffer (50 mM Tris, 100 mM NaCl, 0.5% Triton X-100, 0.5 mM EDTA, 0.15 (w/v) NaN3, 10 mM DTT, pH 7.5) and one time with PBS buffer by sonicating for 10 min, followed by centrifuging at the speed of 12000 g for 10 min each time. In the last step, inclusion bodies were resuspended with P3 buffer (20 mM Tris, 0.5 mM EDTA, 4 M urea, 10 mM DTT, pH 8.0), dissolved overnight while rotating, centrifuged at the speed of 12000 g for 10 min to remove the unsolved particles. The supernatant is the desired denatured protein and was shock frozen and stored at −80 °C until use. 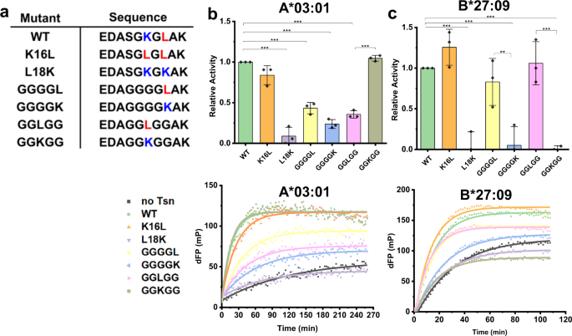Fig. 4: The role of K16 is the F-pocket nature dependent. aThe sequence of Tsn loop11–20mutants. b,cupper panel: Relative activity of tapasin loop11–20mutants to catalyze peptide exchange compared to ERp57-TsnWTtowards A*03:01 and B*27:09. FTIC-KK9 was used for A*03:01, FTIC-IF9 (IRAAKFITCPPLF) was used for better resolution of B*27:09. Error bars (SD) were calculated from three independent experiments. For comparison of loop mutants to WT, the two-sample unequal variance Student’sttest was performed (*p< 0.05, **p< 0.01, ***p< 0.001). Lower panel: Representative peptide exchange profiles of 500 nM A*03:01/photoKK9, and B*27:09/photoRL9 in the absence (black) and presence of equimolar amounts of tapasin loop mutants. dFP means the baseline was subtracted. These curves were recorded on the PerkinElmer VICTOR3V machine. Corresponding heavy chain mutants were generated by standard site directed mutagenesis using heavy chain WT as template, primers used were listed in Supplementary Table 4 . pMHC-I proteins were obtained by refolding heavy chain, β 2 m with high-affinity peptides at 4 °C as described below. Briefly: heavy chain, β2m and the corresponding restricted high-affinity peptide were refolded together in refolding buffer (0.4 M arginine, 0.1 M Tris, GSH:GSSG = 5 mM:0.5 mM, 2 mM EDTA, 0.5 mM PMSF, pH 8.0 for A*03:01 and A*02:01, pH 7.5 for B*27:05/09). For 1 L refolding, 10 mg peptide (photocleavable peptide photoKV9 for A*02:01 first need be dissolved in DMSO) was first added into pre-cooled refolding buffer, followed by dropwise adding 30 mg β2m. After stirring for 2 h at 4 °C, 30 mg heavy chain was dropwise added. The refolding bottle was then kept at 4 °C while stirring (for photocleavable peptides, the refolding bottle need be kept in dark) until purification. The refolding time varies for different allotypes: 3 days for A*02:01, 5 days for A*03:01, 7 days for B*27:09 (heavy chain equipped with or without a His-tag) and B*27:05 without His-tag, 14 days for B*27:05 when heavy chain bears a His-tag. Peptides used for refolding in this study were chemical synthetized (GL Biochem (shanghai) ltd. or DG peptides, China). Peptides’ sequence are also summarized in Supplementary Table 1 : KILGFVFJ*V (photoKV9) for A*02:01, A*02:01Y116D, A*02:01H114D, A*03:01D116Y and A*03:01R114H/D116Y, KLIETYFJ*K (photoKK9) for A*03:01, A*03:01D116Y, A*03:01R114/HD116Y and A*02:01Y116D, RRKWRRWJ*L (photoRL9) for B*27:05/09, B*27:05D116Y and B*27:05H114R, IRAAPPPJ*F (photoIF9) for B*27:05/09, where J* = 3-amino-3-(2-nitrophenyl)-propionic acid [50] , RRKWRRWHL (RL9) for B*27:05/09. Refolded pMHC-I complexes were purified by size-exclusion chromatography (SEC) with a Superdex 200 increase 10/300 GL column in PBS buffer. Pure fractions were pooled, shock frozen and stored at −80 °C until use. The T m of pMHC-I molecules (WT) before and after UV exposure are summarized in Supplementary Table 2 . Expression and purification of ERp57-Tsn mutants and TAPBPR The construct expressing ERp57-Tsn WT was similar as previously described [16] . Briefly, tapasin (1-398) fused with a C-terminal 6xHis-tag was inserted into pFastBac-Dual vector under the polyhedrin promoter between BamH I/ Xba l and ERp57 (1-504, C60A) was inserted under the p10 promotor between Sma I/ Sph I. All scoop loop mutants of ERp57-Tsn were generated by standard site directed mutagenesis using ERp57-Tsn WT as template (unless otherwise stated). Primers used were listed in Supplementary Table 4 . TAPBPR (1-405) fused with a C-terminal 6xHis-tag was inserted into pFastBac1 vector between BamH I and Xba l, C97A mutation was introduced to increase the expression yield of TAPBPR while didn’t affect the activity of TAPBPR [12] . Constructs expressing ERp57-Tsn WT , its mutants and TABPPR were transfected into Sf9 ( Spodoptera frugiperda ) insect cells based on the manufacturer’s protocol (Bac-to-Bac® Baculovirus Expression System, Thermo Fisher) to generate virus stock. Expression of ERp57-Tsn proteins were verified by dot plot with anti-His-tag antibody (anti-His-HRP, dilution 1:2000, Miltenyi Biotec, Mat. No. : 120-003-811, Lot No.:5170502017). Insect cells were harvested 4 days after transfection and cell pellets were lysed in cold lysis buffer (100 mM KH 2 PO 4 , 600 mM KCl, 1% Triton X-100, pH = 8.0). Protease inhibitor, DNase I, MgCl 2 and 5 mM MMTS (MMTS: S-methyl methanethiosulfonate, Sigma-Aldrich, Switzerland, not add when purifying TAPBPR) were freshly added. Supernatant was purified with Protino® Ni-NTA Agarose (Macherey-Nagel™, Germany) by spin column purification method. Briefly, the lysate supernatant (20 ml) was incubated with 0.4 ml buffer equilibrated nickel beads at 4 °C for 30 min–1 h (Ni-NTA Agarose, Macherey-Nagel, Germany) while rotating. Nickel beads were spun down at the speed of 500× g for 5 min and then transferred into a 2-ml eppendorf tube. Nickel beads were washed with 1 ml equilibrium buffer (100 mM KH 2 PO 4 , 600 mM KCl, pH = 8.0) three times and then with 1 ml wash buffer (10 mM imidazole, 100 mM KH 2 PO 4 , 600 mM KCl, pH = 8.0) each time until the A280 absorption lower than 0.2. Protein was eluted with 0.4 ml elution buffer (150 mM imidazole, 100 mM KH 2 PO 4 , 600 mM KCl, pH = 8.0) each time until the A280 absorption below 0.1. Eluted fractions were pooled and further purified by Superdex 200 increase 10/300 GL column in PBS buffer. Purified tapasin mutants and TAPBPR were analyzed by non-reducing 4–12% SDS-PAGE (Supplementary Fig. 5d , also see source data file). Pure fractions were pooled, shock frozen and kept at −80 °C until use. Thermoshift measurements Sypro-orange dye was used to determine the T m of proteins. In all, 20 μl protein (0.2–0.4 mg/ml) was mixed with 5 μl Sypro-orange dilution buffer (243.5 μl buffer + 1.5 μl Sypro-orange, Invitrogen, USA), then added to the MicroAmpROptical 96-well Reaction Plate (Life Technologies), measured on the qPCR machine (Stratagene Mx3005PTM, ThemoFisher) using a protocol with heating at the speed of 2 °C/min from 25 °C to 95 °C. Each sample was measured in three replicates. Experimental data analysis was processed with Origin 2019 and T m was obtained by fitting with the Boltzmann function. NMR chemical shift assignments All NMR spectra (unless otherwise stated) were acquired on a Bruker Avance III 700 MHz spectrometer equipped with a 5-mm triple resonance cryoprobe. Spectra were processed with TopSpin3.2 (Bruker, Billerica, USA) and analyzed with CcpNmr Analysis 2.4.2 [51] . All NMR samples were measured in PBS 7.2 buffer with 10% D 2 O at 300 K (unless otherwise stated). The sequence of B*27:09 heavy chain for preparing NMR samples was the same as the BMRB Entry 25713. In order to confirm backbone amide assignments of the B*27:09 heavy chain, B*27:09 heavy chain was isotope-labeled with 15 N, 13 C, and 2 H. For 1 L deuterated M9 medium culture, 1 g 15 NH 4 Cl and 1.5 g d -glucose-U- 13 C6,1,2,3,4,5,6,6-d7 (Cambridge Isotope Laboratories, Inc.) were used. The inclusion body was then purified in protonated buffer to allow for 1 H- 15 N-detection. The backbone amide assignments of B*27:09 heavy chain were transferred from available assignments for B*27:09/RL9 (BMRB Entry 25713) and confirmed with HNCA, HNCO, and 1 H- 15 N-TROSY-HSQC spectra with 15 N- 13 C- 2 H B*27:09/RL9 (270 μM). 1 H- 15 N-TROSY-HSQC spectrum of 2 H- 15 N B*27:09/photoRL9 was recorded at a concentration of 250 μM and the assignments were transferred from the confirmed assignments of 15 N- 13 C- 2 H B*27:09/RL9 (Supplementary Fig. 9 ). In order to investigate methyl-group dynamics of B*27:09, Ile, Val, and Leu methyl groups were 1 H- 13 C labeled in a deuterated 15 N/ 12 C background. For 1 L deuterated M9 medium culture, 100 mg precursor for Val and Leu (2-keto-(3-methyl- 13 C)-butyric-4- 13 C,3-d acid sodium salt, Santa Cruz Biotechnology, Inc) and 50 mg precursor for Ile (2-ketobutyric acid-4− 13 C,3,3-d2 sodium salt hydrate, Sigma-Aldrich, USA), 1.5 g 15 NH 4 Cl and 1.5 g d -glucose-U- 12 C6,1,2,3,4,5,6,6-d7 were added. ILV methyl assignments were obtained with a {I( 13 CH 3- only), L( 13 CH 3 , 12 CD 3 ), V( 13 CH 3 , 12 CD 3 )} U-[ 15 N, 13 C, 2 H] sample of B*27:09/RL9 at 310 K, using a HMCM[CG]CBCA spectrum [52] acquired at a Bruker AV-III 600 spectrometer using a TCI-cryoprobe equipped with one-axis self-shielding gradients. The sample had a concentration of 26 mg/ml in 10 mM phosphate pH 7.5, 150 mM NaCl, and 10% D 2 O and methyl assignments are updated in BMRB entry 25713. These assignments as well as those available for A*02:01 (BMRB Entry 27631) and A*01:01 (BMRB Entry 27632) were used to transfer assignments to other complexes used in this publication [30] . Transferred assignments were validated where possible by methyl-methyl and methyl-amide NOEs with 170 µm 1 H- 13 C-ILV- 15 N- 2 H B*27:05/photoRL9 in combination with the crystal structure of B*27:05/RL9 (PDB ID 1OGT). The 1 H- 13 C HSQC spectra of B*27:09/RL9 and B*27:09/photoRL9 are shown in Supplementary Fig. 9 . CPMG relaxation dispersion Carr-Purcell-Meiboom-Gill (CPMG) relaxation dispersion experiments of 150 μM ~ 250 μM 1 H- 13 C-ILV- 15 N- 2 H B*27:09/photoRL9 were recorded single-scan interleaved using an INEPT transfer for excitation [53] and a WATERGATRE element for water suppression in order to measure in 10% D 2 O. CPMG pulse frequencies of 0, 950, 50, 300, 150, 800, 100, 250, 400, 600, 200, 50, 500, 300, and 700 with a constant time delay of 40 ms were used. Peak intensities were converted to the \({R}_{2}^{{{\mathrm{eff}}}}\) transverse decay rates with the equation \({R}_{2}^{{{\mathrm{eff}}}}=1/{T}_{{{\mathrm{CPMG}}}}\times {\rm{ln}}({I}_{0}/{I}_{{{\mathrm{CPMG}}}})\) . Only assigned peaks were analyzed. CPMG profiles of all methyl groups displaying dispersion ( \({R}_{2}^{{{\mathrm{eff}}}}\) > 2 s -1 ) were fitted to a two-state model using the program NESSY [54] . HSQC spectra after UV exposure and in the presence of ERp57-Tsn 1 H- 15 N-TROSY-HSQC spectra of 50 µM 1 H- 13 C-ILV- 15 N- 2 H B*27:09/photoRL9 were recorded before and after UV exposure. Peak intensity ratios (I/I0) were calculated from spectra before (I0) and after (I) UV exposure. In order to study how B*27:09/photoRL9 would be affected by tapasin in solution, 1 H- 15 N-TROSY-HSQC spectra of 50 μM 1 H- 13 C-ILV- 15 N- 2 H B*27:09/photoRL9 in the absence (I0) and presence (I) of 50 μM un-labeled ERp57-Tsn WT purified in matched buffer (PBS 7.2) were recorded and peak intensity ratios (I/I0) were calculated. Fluorescence Polarization assay Peptide exchange assays of MHC-I were done with UV-exposed MHC-I refolded with photocleavable peptide (photo-MHC-I) exchanging against FITC-labeled high-affinity peptides in the absence or presence of ERp57-Tsn WT , its mutants or TAPBPR. All proteins used were purified in the same buffer (PBS pH 7.4, unless otherwise stated). Briefly: 20 μl of a 1 μM purified photo-MHC-I was UV exposed (arc-UV lamp, Newport 6295NS, filter 345 nm, 1000 W) on ice for 5 min at a distance of 15 cm and then added to the 384-well assay plate (Corning® 384-well Low Flange Black Flat Bottom Polystyrene NBS Microplate 3575, USA). In total, 10 μl of a 2 μM ERp57-Tsn WT or mutants or 10 μl PBS buffer were added and then 10 μl of a 40 nM corresponding FITC-peptide were added right before measurement. Wells containing only FITC-peptide (final 10 nM) were measured as baseline. Each well has a total volume of 40 μl and experiment was performed at room temperature with three replicates. FP signals were recorded on PerkinElmer VICTOR 3 V (Fig. 4b , Supplementary Fig. 1a , and Supplementary Fig. 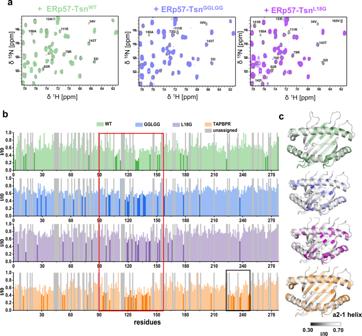Fig. 5: NMR analysis of tapasin mutants interacting with MHC-I. aRepresentative zoom view of the overlay of1H-15N TROSY-HSQC spectra of 50 µM B*27:09/photoRL9 (gray) and in the presence of equimolar ERp57-TsnWT(green), ERp57-TsnGGLGG(blue) or ERp57-TsnL18G(purple). Attenuated peaks are marked.bPeak intensity ratio analysis (I/I0) of B*27:09/photoRL9 in the presence of ERp57-TsnWT, ERp57-TsnL18G, ERp57-TsnGGLGG, and TAPBPR against B*27:09/photoRL9 (I0) are plotted against residue sequence. Significantly reduced residues (below I/I0 average – δ) were highlighted in corresponding dark color. Unassigned residues are plotted as gray bars. Red squared region means affected region in the peptide binding groove in the presence of tapasin or TAPBPR. Black squared region means region only affected by TAPPBR.cPeak intensity ratio (I/I0) are mapped as B-factor on the structure of B*27:09. The range of the intensity ratio is from 0.3 to 0.7 for all mutants. The color code is the same as inb. Unassigned residues are plotted as white color. 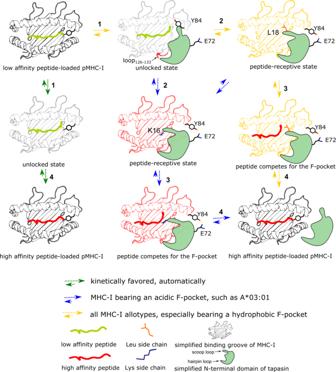Fig. 6: The proposed mechanism of tapasin-mediated peptide exchange. Step 1: pMHC-I molecules sample conformations, which determine peptide binding and tapapsin binding. Tapasin recognizes a certain state of pMHC-I by approaching pMHC-I from the α2-helix side of the pMHC-I. Interaction between its loop187-196with the loop126-133of heavy chain provides initial binding which alters the dynamics of the peptide binding groove and subsequently together with the interaction between its E72 in strands β3 and Y84 of the heavy chain promote the C-terminus of peptide to adopt loose binding in the F-pocket accompanied. Now pMHC-I switches to the unlocked state. MHC-I charged with very low affinity peptide can switch to peptide unlocked state automatically by the motion of the bound peptide adopting loose binding state. Step 2: The scoop loop11-20interacts with the F-pocket region and stabilize the F-pocket with side chain of L18. Now pMHC-I switches to the peptide receptive state. For allotypes bearing a negatively charged F-pocket, tapasin can also use the residue K16 in the scoop loop11-20to stabilize the charged F-pocket, which increases the efficiency of tapasin-mediated peptide exchange. Step 3: The upcoming peptide competes for the F-pocket until the affinity is high enough to replace the side chain. Step 4: Once the high-affinity peptide binds, tapasin is released from the pMHC-I. 2 ) or recorded on Tecan Spark plate reader (Figs. 2b and 3b and Supplementary Fig. 4 ) with an excitation filter of λ ex =  485 nm and an emission filter of λ em = 535 nm and monitored over time range from 1 to 5 h. FITC-labeled high-affinity peptides used in this study are GILG-Lys FITC VFTV for A*02:01, KILG-Lys FITC VFTV for A*02:01, A*02:01Y116D, KLIE-Lys FITC YFSK for A*03:01, KLIE-Lys FITC YFSV for A*03:01D116Y, A*03:01R114HD116Y, A*02:01, and A*02:01Y116D, RRKW-Lys FITC RWHL for B*27:05/09, B*27:05D116Y and B*27:05H114R, and IRAA-Lys FITC PPLF for B*27:05/09 (summarized in Supplementary Table 1 ). Experimental data analysis was processed with Origin 2019 and the observed association rate K on was calculated by using fitting function \(Y={Y}_{0}-A{e}^{-{Kt}}\) , where Y 0 is the maximum value and A is the increased FP range. X-ray crystallography Sample for crystallography was purified two times by SEC in 20 mM Tris/HCl pH 7.4, 150 mM NaCl, 0.01% sodium azide, and concentrated to 13–15 mg/ml as measured by the absorbance at 280 nm. Crystals were obtained by the sitting-drop vapor-diffusion method at 18 °C with a reservoir solution composed of 20% (w/v) polyethylene glycol 3350, and 200 mM KSCN. Crystal growth and diffraction quality was improved by microseeding. Prior to flash cooling of the crystals in liquid nitrogen, glycerol was added to the mother liquor to a final concentration of 25% (w/v). Synchrotron diffraction data were collected at the beamline 14.1 of the MX Joint Berlin laboratory at BESSY II (Berlin, Germany). X-ray data collection was performed at 100 K. Diffraction data were indexed and processed with the XDS. Data collection and refinement statistics are given in supplementary Table 1 . The phase problem was solved by molecular replacement using the program PHASER [55] with the structure of HLA-B*27:09/pVIPR as search model (PDB ID 5IB5 [56] ). The structure was initially refined by applying a simulated annealing protocol and in later refinement cycles by maximum-likelihood restrained refinement using in PHENIX [57] , [58] . Model building and water picking was performed with COOT [59] . Intermediate and final structures were evaluated with and MOLPROBITY [60] and the JCSG validation server (JCSG Quality Control Check v3.1). Figures were prepared with PyMOL (Version 1.8 Schrödinger, LLC). Atomic coordinates and structure factor amplitudes have been deposited in the Protein Data Bank under accession code 7ALO. Mass-spectrometric analysis UV-exposed photo-MHC-I was purified by SEC to remove any possible fragment. In order to detect fragments of the photocleavable peptide, SEC fractions were analyzed by matrix-assisted laser desorption ionization-time of flight mass spectrometry (MALDI-TOF-MS) using α-cyano-4-hydroxycinnamic acid (HCCA) as matrix. The samples were applied on the MALDI target using the dried-droplet technique. Spectra were recorded on an Ultraflex-II TOF/TOF instrument (Bruker Daltonics, Bremen, Germany) in the positive reflector mode in the m / z range of 600–4000. Samples of photocleavable peptide before and after UV exposure served as a reference. Modeling of the tapasin scoop loop The EM structure of the PLC, PDB ID 6ENY) served as a scaffold to build the MHC-I-ERp57-Tsn models using the crystal structures of MHC- I allotypes HLA-A*02:01 (PDB ID 1OGA), HLA-A*03:01 (PDB ID 2XPG), HLA-B*27:05 (PDB ID 1OGT), HLA-B*27:09 (PDB ID 1OF2), and the ERp57-Tsn complex (PDB ID 3F8U). The unresolved atoms in the tapasin scoop loop were modeled and refined with the MODELLER software [61] , [62] using the corresponding sequence to generate an ensemble of 100 models for each allotype. With the Amber 12 simulation package, each MHC-I-ERp57-Tsn model was placed in an octahedral TiP3 [63] , [64] , [65] water box and neutralized with counterions. Then, each complex was energy minimized, positionally restrained (25 kcal mol −1 Å −2 ), and heated from 100 to 300 K. The restraints were resolved in five steps, and then each complex was equilibrated for 2 ns. Short-range nonbonded interactions were taken into account up to a cut-off value of 9 Å. Modeling and scoring of tapasin mutants The structural modeling of the tapasin mutants was performed with PyRosetta using the “ref2015” energy function [43] , [44] , [45] . The desired scoop loop sequence was computationally introduced into tapasin, followed by Monte Carlo-based simulated annealing sidechain and backbone minimization steps. The energy scores were calculated with the “score_jd2” application and averaged for all generated models per mutant. Reporting summary Further information on research design is available in the Nature Research Reporting Summary linked to this article.